Regulation of focal adhesion formation by a vinculin-Arp2/3 hybrid complex Focal adhesions (FAs) are large multi-protein complexes that act as transmembrane links between the extracellular matrix and the actin cytoskeleton. Recently, FAs were extensively characterized, yet the molecular mechanisms underlying their mechanical and signalling functions remain unresolved. To address this question, we isolated protein complexes containing different FA components, from chicken smooth muscle, and characterized their properties. Here we identified ‘hybrid complexes’ consisting of the actin-nucleating subunits of Arp2/3 and either vinculin or vinculin and α-actinin. We further show that suppression of p41-ARC, a central component of native Arp2/3, which is absent from the hybrid complexes, increases the levels of the Arp2/3-nucleating core in FA sites and stimulates FA growth and dynamics. In contrast, overexpression of p41-ARC adversely affects FAs. These results support the view that Arp2/3 can form modular ‘hybrid complexes’ containing an actin-nucleating ‘functional core’, and ‘anchoring domains’ (vinculin/p41-ARC) that regulate its subcellular localization. Focal adhesions (FAs) are micrometer-scale subcellular structures that mediate the interactions of cells with the underlying extracellular matrix (ECM) and anchor the actin cytoskeleton to their cytoplasmic aspects [1] , [2] , [3] , [4] , [5] , [6] . These adhesions contain clusters of transmembrane integrin receptors that bridge between the extracellular matrix and the termini of actin stress fibres [7] , [8] , [9] via a network of proteins, collectively referred to as the ‘integrin adhesome’. The adhesome consists of a wide variety of integrin receptors, signalling molecules, actin-associated and adapter proteins that participate in the regulation of FA formation, turnover and signalling [10] . Overall, these adhesive structures participate in many key processes, including cellular and tissue morphogenesis, cell migration, division, survival and differentiation [11] , [12] , [13] , [14] . The mechanism by which the integrin adhesome, with its 200 or so tightly interconnected components ( http://www.adhesome.org ) [15] , takes part in these complex processes is still poorly understood. Nevertheless, recent insights into the functional architecture of FAs were obtained, using correlative light/cryo-electron tomography [16] and 3D super-resolution fluorescence microscopy [17] . These studies indicated that integrin adhesions are laminated structures in which actin filaments interact with distinct membrane-associated particles [16] , and that different FA proteins are spatially ordered at the membrane–cytoskeleton interface [17] . Advanced proteomics, combined with protein crosslinking, provided further information, suggesting a hierarchy of molecular interactions within integrin adhesions, which are modulated in response to different experimental perturbations [18] , [19] , [20] . In this study, we combined biochemical approaches with native mass spectrometry (MS) and cellular biology, in an attempt to explore the mechanism underlying actin polymerization at FA sites. Our strategy was to isolate and characterize complexes that are associated with FAs and contain actin-polymerizing components. We chose chicken smooth muscle, which is particularly enriched with adhesome proteins as our source for such complexes. Here we show that several novel multi-protein complexes are present in smooth muscle extracts, prominent among them, are complexes containing vinculin, or vinculin and α-actinin, bound to Arp2/3 subunits. The isolation and characterization of which will be addressed below. Formins and Arp2/3 were previously suggested to act at local nucleation sites of actin polymerization in FAs [21] , [22] , [23] , [24] , [25] , [26] . Formins are a large family of FH1 domain-containing dimeric proteins, capable of actin nucleation and processive movement on the filaments’ barbed ends. Thus, formins create and elongate new linear actin filaments [27] . Specifically, the formins mDia1 and 2 and Formin 1 isoform IV have been shown to be required for the formation of FAs and have the capacity to modulate their characteristics, whereas FHOD1 has been shown to localize into early adhesion sites [26] , [28] , [29] , [30] . In contrast, the Arp2/3 complex is mostly known for its ability to drive a branching polymerization of actin filaments [31] . Both Arp2 and Arp3, its two actin-related subunits, function as a template for the initiation of a new actin filament that branches off from an existing network [32] , [33] . Although the intact Arp2/3 complex contains seven subunits, Arp3, Arp2, p41-ARC, p34-ARC, p21-ARC, p20-ARC and p16-ARC, only Arp3, Arp2 and p34-ARC are considered to be directly involved in the polymerization process [34] , [35] . The exact role of the other four subunits is less clear: p21-ARC is thought to regulate the efficiency of actin nucleation [34] and promote persistent chemotactic cell migration [36] ; p20-ARC is suspected to have a structural role in holding p16-ARC and p41-ARC in the complex [34] , [35] , and p41-ARC is believed to target the intact complex to the parent filament [37] . Previous studies indicated that Arp2/3 can interact temporarily with vinculin and FA kinase [38] , [39] and associate with crosslinked integrin complexes [18] . However, despite these findings, the mode of interaction of Arp2/3 with FAs, and its biological role in FA formation, is still unclear. In this work, we characterized one set of stable protein complexes isolated from smooth muscle tissue, which contain vinculin, associated with the actin-nucleating core of Arp2/3 with or without α-actinin. Our results indicate that knockdown of p41-ARC, an Arp2/3 subunit that is not incorporated into either of the two complexes, leads to elevated Arp2/3 levels in FAs of cultured cells and induces the formation of large and dynamic FAs. In contrast, overexpression of p41-ARC markedly suppressed FA formation. These results are in line with the hypothesis that Arp2/3 has a modular structure, whereby its functional (actin nucleating) core (that is, Arp2, Arp3, p34-ARC) can associate with different anchoring molecules (for example, p41-ARC or vinculin) that direct its subcellular localization to different subcellular sites, such as lamellipodia or FAs, respectively. Purification of FA-associated protein complexes As a source for the isolation of FA-associated protein complexes, we used chicken gizzard smooth muscle. During the past several decades, this tissue has been successfully used for the purification of adhesion-related and cytoskeletal proteins including vinculin, paxillin, talin and α-actinin [40] , [41] , [42] , [43] , [44] . Careful examination of the purification procedures described in these early studies indicates that multiple proteins tend to coelute during gel filtration chromatography, and their dissociation from each other occurs on treatment with high salt concentrations or exposure to denaturing conditions. These findings suggested that multi-protein complexes may exist in gizzard tissue, which may remain intact on extraction under close to native conditions. To effectively isolate intact protein complexes while removing the vast amounts of actin and myosin, we employed a stepwise extraction protocol utilizing a high concentration of ATP to dissociate the actomyosin filaments, followed by short incubation of the pellet at pH=9.0 at 37 °C to solubilize the FA-associated components ( Fig. 1a ). The extracted proteins were further concentrated and fractionated using ammonium sulphate precipitations followed by gel filtration on Sepharose 4B, capable of separating proteins and protein complexes within the range of 0.1–10.0 MDa (for details, see Methods, and Fig. 1a ). Monitoring the absorbance of proteins in the eluate at 280 nm revealed several distinct peaks, each of which contained multiple proteins (for example, talin, α-actinin, vinculin and metavinculin) with wide variations in mass, suggesting that they might be components of multi-protein complexes ( Fig. 1b ). 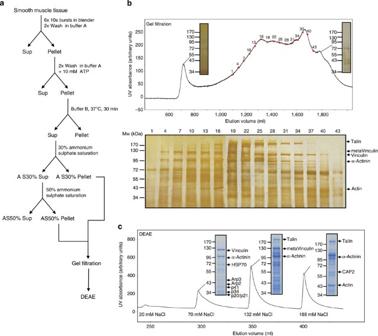Figure 1: Purification of adhesion-related protein complexes. (a) Workflow of the purification procedure. (b) Size-exclusion gel filtration chromatogram and SDS-PAGE analysis of the eluted fractions. Numbered red dots represent corresponding fractions in the SDS-PAGE analysis. (c) Chromatography pattern of the stepwise elution from the DEAE column and SDS-page analysis of protein fractions. Figure 1: Purification of adhesion-related protein complexes. ( a ) Workflow of the purification procedure. ( b ) Size-exclusion gel filtration chromatogram and SDS-PAGE analysis of the eluted fractions. Numbered red dots represent corresponding fractions in the SDS-PAGE analysis. ( c ) Chromatography pattern of the stepwise elution from the DEAE column and SDS-page analysis of protein fractions. Full size image Despite the effective separation of protein complexes, achieved by this gel filtration column, protein peaks were overlapping and were not sufficiently pure to be directly examined by native MS. Therefore, we collected the main peak containing various prominent adhesome components, loaded it onto a DEAE-Sepharose column and conducted a stepwise elution, maintaining near-physiological buffer conditions throughout the process (a typical elution chromatogram and representative gel band patterns are shown in Fig. 1c ). The first DEAE-Sepharose fraction, eluted at 70 mM NaCl, was further subjected to proteomic MS analysis, indicating that its major constituents are vinculin, α-actinin and all seven subunits of the Arp2/3 protein complex. Characterization of this fraction is described below. Vinculin interacts with the functional core of Arp2/3 As a basic prerequisite for unambiguous native MS analysis, we had to obtain the precise masses of all protein components in this fraction. This was accomplished by combining MS-based proteomic identification of proteins extracted from gel bands, structural MS/MS analysis and a monolithic column-based approach. In brief, the monolithic column was used under denaturing conditions to separate the individual subunits of the isolated complexes [45] . The eluted flow from this column was split, using a Nanomate robot (see Methods). One fraction was sprayed directly into the mass spectrometer for accurate mass determination, while the second was collected for sequence identification following tryptic digestion, MS analysis and a database search [45] . This approach enabled us to relate the specific subunit sequences with the accurate masses (see Table 1 for subunit masses and identities). Table 1 Theoretical and measured masses of individual proteins and protein complexes. Full size table The composition of the vinculin-containing protein complexes was then investigated by applying native MS and MS/MS approaches under conditions that preserve non-covalent interactions [46] . An electrospray mass spectrum revealed four different charge series ( Fig. 2a ). The major charge state, centred at ~5,800 m/z , corresponded in mass to free vinculin. The remaining charge states overlapped in the region of 7,000 to 11,000 m/z . The highly abundant species had an experimental mass of 262,620±39 Da (where ± represents the mass measurement error), while the remaining minor series corresponded to 223,452±6 Da and 345,681±41 Da. On the basis of the assigned unique mass of each of the proteins ( Table 1 ) and the use of the ‘SUMMIT’ algorithm, which calculates all possible protein compositions that add up to the target mass within a given error range [47] , the composition of the complexes could be unambiguously assigned. The masses measured suggest the presence of three different protein complexes corresponding to vinculin-Arp2-Arp3-p21-p34 (Vin-Arp), intact Arp2/3 and vinculin-α actinin-Arp2-Arp3-p34 (Vin-αAct-Arp), respectively. 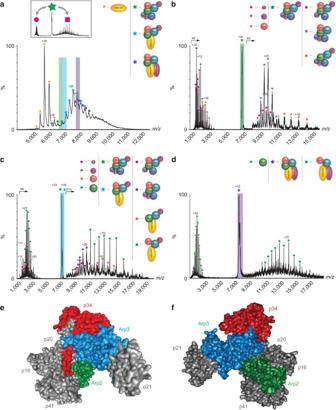Figure 2: Multiple forms of the Arp2/3 complex coexist. (a) Mass spectrum of the 70 mM fraction isolated from the DEAE column and recorded under native conditions. The predominant species detected, within the range of 5,000–6,800m/z, is assigned to monomeric vinculin. Additional charge states, which correspond in mass to three coexisting protein complexes, are observed between 7,000 and 11,000m/z. The masses of these complexes indicate the presence of intact Arp2/3, a vinculin-associated Arp2/3 complex and a vinculin-α actinin-associated Arp2/3 complex. Validation of the complexes’ composition was undertaken by means of tandem MS; selected charge states are shaded in green, blue and purple, respectively. The inset exemplifies the labeling of the MS/MS spectra inb–d. The isolated peak is labeled with a star. Circles denote the released subunits and squares correspond to the remaining stripped complex. (b) MS/MS spectrum showing the dissociation products of ions isolated at 6,917m/z. Charge states above 7,000m/zcorrespond to ‘stripped’ Arp2/3 complexes. Individual Arp2/3 subunits, p16, p21 and p34 are observed at the lowm/zvalues. On the basis of an analysis of the spectrum, we could conclude that Arp2/3 is detected in the sample. Similarly, we deduced that the charge states selected incanddcorrespond to the existence of a vinculin, Arp2, Arp3, p34-ARC, p21-ARC complex, and a vinculin+α actinin, Arp2, Arp3, p34-ARC complex. (e,f) Two views of the surface representation of the Arp2/3 complex rotated by approximately 180° (PDB entry 1K8K). Subunits that are part of the Vin-Arp or the Vin-αAct-Arp complexes are denoted according to the colour scheme described above (a–d), while the remaining subunits are shown in grey (p21 which is part of Vin-Arp and not Vin-αAct-Arp is also coloured in grey). The coloured surfaces highlight the neighbouring positions of the ‘functional core’ subunits of Arp2/3. Figure 2: Multiple forms of the Arp2/3 complex coexist. ( a ) Mass spectrum of the 70 mM fraction isolated from the DEAE column and recorded under native conditions. The predominant species detected, within the range of 5,000–6,800 m/z , is assigned to monomeric vinculin. Additional charge states, which correspond in mass to three coexisting protein complexes, are observed between 7,000 and 11,000 m/z . The masses of these complexes indicate the presence of intact Arp2/3, a vinculin-associated Arp2/3 complex and a vinculin-α actinin-associated Arp2/3 complex. Validation of the complexes’ composition was undertaken by means of tandem MS; selected charge states are shaded in green, blue and purple, respectively. The inset exemplifies the labeling of the MS/MS spectra in b – d . The isolated peak is labeled with a star. Circles denote the released subunits and squares correspond to the remaining stripped complex. ( b ) MS/MS spectrum showing the dissociation products of ions isolated at 6,917 m/z . Charge states above 7,000 m/z correspond to ‘stripped’ Arp2/3 complexes. Individual Arp2/3 subunits, p16, p21 and p34 are observed at the low m/z values. On the basis of an analysis of the spectrum, we could conclude that Arp2/3 is detected in the sample. Similarly, we deduced that the charge states selected in c and d correspond to the existence of a vinculin, Arp2, Arp3, p34-ARC, p21-ARC complex, and a vinculin+α actinin, Arp2, Arp3, p34-ARC complex. ( e , f ) Two views of the surface representation of the Arp2/3 complex rotated by approximately 180° (PDB entry 1K8K). Subunits that are part of the Vin-Arp or the Vin-αAct-Arp complexes are denoted according to the colour scheme described above ( a – d ), while the remaining subunits are shown in grey (p21 which is part of Vin-Arp and not Vin-αAct-Arp is also coloured in grey). The coloured surfaces highlight the neighbouring positions of the ‘functional core’ subunits of Arp2/3. Full size image To confirm the identities of the coexisting protein complexes, we employed the tandem MS approach. In this type of experiment, a specific well-defined m/z range that includes the parent ion is selected and accelerated into an argon-filled cell to induce its activation. As a result, individual highly charged subunits are dissociated from the parent ion, producing ‘stripped’ complexes with charge states lower than that of the original ion. This sequential removal of highly charged monomers leads to an effective charge reduction in the parent ions, such that the composition and stoichiometry of the complex can be unambiguously identified [48] . In this way, three MS/MS experiments were carried out, and a parent ion corresponding to each of the three complexes was selected ( Fig. 2b–d and Supplementary Fig. 1 ). From the analysis of the dissociation patterns, that is, measuring the masses of the individual subunits observed at the low- m/z region and their corresponding ‘stripped complexes’, we concluded that Vin-Arp, intact Arp2/3 and Vin-αAct-Arp coexist simultaneously in the sample. Our data indicate that vinculin is associated only with the functional core of Arp2/3, but not with the intact complex. The reproducibility of the results and the fact that the intact Arp2/3 complex, but no free subunits, was detected in the MS spectra render it unlikely that Arp2/3 is dissociated during the purification process, leading to a non-physiological association of its subunits with vinculin and α-actinin. To further consolidate these results, using an independent experimental approach, we performed protein extraction from fresh gizzards under close to native conditions and found that vinculin coimmunoprecipitates along with Arp3 ( Fig. 3a ). Moreover, even before the size exclusion and ion exchange chromatography steps we could detect three p34-ARC-containing bands in native gel electrophoresis, of which, as expected, only two were vinculin positive ( Fig. 3b ). Thus, the Vin-Arp complexes seem to be genuine and not purification artefacts. Furthermore, examination of the Arp2/3 crystal structure ( Fig. 2e,f ) supports our observations, as Arp2, Arp3, p34-ARC and p21-ARC are found to be in tight contact with one another. 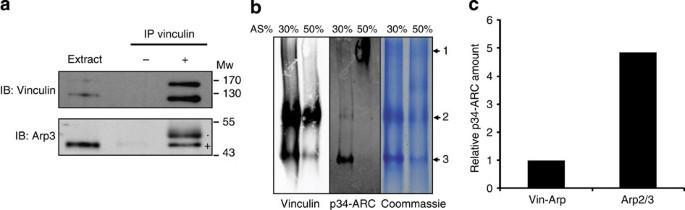Figure 3: The relative abundance of the Vin-Arp and Vin-αAct-Arp in chicken gizzard extracts. (a) Immunorecipitation of vinculin, metavinculin and Arp3 from gizzard extracts at pH=8.0 indicated that vinculin and Arp2/3 interact in chicken gizzard extracts. The dot is IgG heavy chain and the plus is Arp3. The original western blot is presented inSupplementary Fig. 5a. (b) Native gel analysis of 30 and 50% ammonium sulphate saturated fractions, blotted against vinculin p34-ARC or coommassie stained. (c) Quantification of p34-ARC band intensity from the native gel. Figure 3: The relative abundance of the Vin-Arp and Vin-αAct-Arp in chicken gizzard extracts. ( a ) Immunorecipitation of vinculin, metavinculin and Arp3 from gizzard extracts at pH=8.0 indicated that vinculin and Arp2/3 interact in chicken gizzard extracts. The dot is IgG heavy chain and the plus is Arp3. The original western blot is presented in Supplementary Fig. 5a . ( b ) Native gel analysis of 30 and 50% ammonium sulphate saturated fractions, blotted against vinculin p34-ARC or coommassie stained. ( c ) Quantification of p34-ARC band intensity from the native gel. Full size image Quantitative analysis of the native gel bands indicates that the relative amount of Vin-Arp and Vin-αAct-Arp is significantly lower than that of the ‘classical’ Arp2/3 ( Fig. 3b,c ). Moreover, in comparison with the Arp2/3 complex, the vinculin hybrid complexes have decreased stability, as exposure to 1 M ammonium acetate induced dissociation of these complexes ( Fig. 4 ). Overall, these observations might explain why these vinculin-Arp2/3 hybrid complexes escaped previous identification. 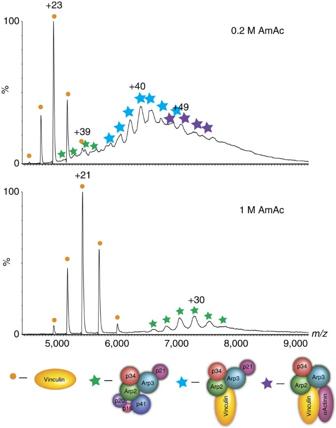Figure 4: Stability of the vinculin-Arp2/3 hybrid complexes. Native MS analysis of the 70 mM NaCl eluted DEAE fraction in the presence of 200 mM ammonium acetate or 1,000 mM ammonium acetate. Figure 4: Stability of the vinculin-Arp2/3 hybrid complexes. Native MS analysis of the 70 mM NaCl eluted DEAE fraction in the presence of 200 mM ammonium acetate or 1,000 mM ammonium acetate. Full size image Possible role for the hybrid complexes in FA formation The findings presented above raise the possibility that Arp2/3 might partner with other molecules (vinculin or vinculin and α-actinin, in our case), thereby affecting their mode or site of action (for example, modulating FA formation). One attractive hypothesis was that the ‘functional core module’ of Arp2/3, which is responsible for actin nucleation, might bind, alternatively, to different ‘anchoring modules’ that direct the actin polymerization activity to different subcellular sites (for example, the lamellipodium or FAs). To test this hypothesis, we knocked down each one of Arp2/3’s seven subunits in HeLa cells using short interfering RNA (siRNA) duplexes and tested the effect of this perturbation on FAs and F-actin organization ( Fig. 5a,b and Supplementary Fig. 2 ). 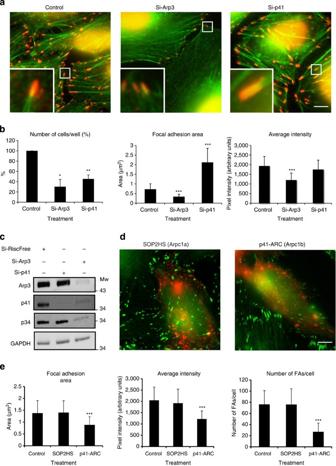Figure 5: Knockdown of Arp3 and p41-ARC exerts opposite effects on FAs and stress fibres. (a) Staining of HeLa cells transfected with siRNA directed against Arp3 and p41-ARC, with vinculin antibodies and phalloidin (used for visualization of F-actin). Scale bar, 10 μm. (b) Quantification of different FA and cell parameters: 20 cells were quantified for each treatment. Focal adhesion area and pixel intensity values represent the 90th percentile, while the number of FAs per cell and the number of cells per well are averaged values. Bars represent ±s.d. *P<0.05, **P<0.005, ***P<0.0005,P-values were calculated by a two-tailed Studentt-test. (c) Validation of siRNA function and its influence on subunit abundance is examined by western blot analysis. The original western blot is presented inSupplementary Fig. 5b. (d) Staining of zyxin, a FA marker, and the myc epitope in HeLa cells overexpressing p41-ARC-myc or SOP2HS-myc. Scale bar, 10 μm. (e) Quantification of different FA and cell parameters: 20 cells were quantified for each treatment. FA area, number and pixel intensity values represent the 90th percentile, while the numbers of FAs per cell are averaged values. Bars represent ±s.d. Figure 5: Knockdown of Arp3 and p41-ARC exerts opposite effects on FAs and stress fibres. ( a ) Staining of HeLa cells transfected with siRNA directed against Arp3 and p41-ARC, with vinculin antibodies and phalloidin (used for visualization of F-actin). Scale bar, 10 μm. ( b ) Quantification of different FA and cell parameters: 20 cells were quantified for each treatment. Focal adhesion area and pixel intensity values represent the 90th percentile, while the number of FAs per cell and the number of cells per well are averaged values. Bars represent ±s.d. * P <0.05, ** P <0.005, *** P <0.0005, P -values were calculated by a two-tailed Student t -test. ( c ) Validation of siRNA function and its influence on subunit abundance is examined by western blot analysis. The original western blot is presented in Supplementary Fig. 5b . ( d ) Staining of zyxin, a FA marker, and the myc epitope in HeLa cells overexpressing p41-ARC-myc or SOP2HS-myc. Scale bar, 10 μm. ( e ) Quantification of different FA and cell parameters: 20 cells were quantified for each treatment. FA area, number and pixel intensity values represent the 90th percentile, while the numbers of FAs per cell are averaged values. Bars represent ±s.d. Full size image Examination of the treated cultures indicated that knockdown of each of the Arp2/3 subunits resulted in a conspicuous reduction in the number of adherent cells, compared with short interfering RNA-induced silencing complex free (siRISC) transfected or untreated cells. Nevertheless, checking the residual cells, only Arp3 and p41-ARC knockdown induced major changes in vinculin, F-actin and Arp2 distribution ( Figs 5a,b and 6a ). Knocking down Arp3 induced major disarray in F-actin organization, accompanied by a reduction in FA number, size and fluorescence intensity of vinculin. Given that Arp3 is considered to be essential for Arp2/3’s actin-nucleating activity, this observation was not surprising. Furthermore, knockdown of Arp3, which lies within the core of the complex and is crucial for its structural integrity, reproducibly induces reduction in the levels of other Arp2/3 subunits such as p41-ARC and p34-ARC ( Fig. 5c and (ref. 34 )). 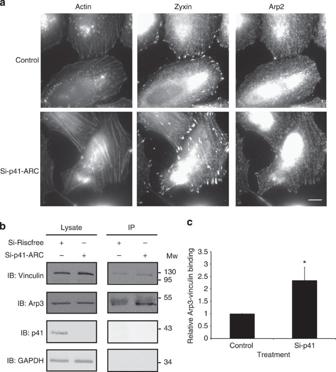Figure 6: p41-ARC knockdown induces increased recruitment of Arp2/3 complexes into FAs by vinculin. (a) Staining for actin with phalloidin, FAs with zyxin and Arp2 in control and p41-ARC knockdown cells. Scale bar, 10 μm. (b) Immunoblotting analysis of co-immunoprecipitation assays in HeLa cells using vinculin-directed antibodies. Plus indicates Arp3 and the dot marks IgG background. The full scanned western blot is presented inSupplementary Fig. 5c. (c) Quantification of CO-IP from three different experiments by western blot. *P<0.05,P-values were calculated by a two-tailed Studentt-test. Various antibody concentrations and exposures were performed to ensure that p41 is absent from the anti-vinculin co-immunoprecipitation. Figure 6: p41-ARC knockdown induces increased recruitment of Arp2/3 complexes into FAs by vinculin. ( a ) Staining for actin with phalloidin, FAs with zyxin and Arp2 in control and p41-ARC knockdown cells. Scale bar, 10 μm. ( b ) Immunoblotting analysis of co-immunoprecipitation assays in HeLa cells using vinculin-directed antibodies. Plus indicates Arp3 and the dot marks IgG background. The full scanned western blot is presented in Supplementary Fig. 5c . ( c ) Quantification of CO-IP from three different experiments by western blot. * P <0.05, P -values were calculated by a two-tailed Student t -test. Various antibody concentrations and exposures were performed to ensure that p41 is absent from the anti-vinculin co-immunoprecipitation. Full size image In sharp contrast to Arp3, knockdown of p41-ARC induced major enhancement of both stress fibre assembly and FA formation. The stress fibres formed in the knocked down cells were over twofold thicker than those found in untreated cells or cells transfected with non-targeting duplexes ( Fig. 5a,b ). The FAs in the knocked down cells (labelled for vinculin) were also considerably larger than those of controls ( Fig. 5a,b ). Live cell monitoring of FA organization indicated that the FAs formed by these cells were not only just larger but also considerably more dynamic than those of control cells, displaying apparent centripetal ‘sliding’, growth and disassembly (Supplementary Movie 1). In contrast, overexpression of p41-ARC had the opposite effect, strongly suppressing FA formation, leading to small and faint adhesions. Interestingly, overexpression of SOP2HS, a variant of p41-ARC, displayed a different subcellular distribution and had no apparent effect on FA assembly ( Fig. 5d,e and Supplementary Fig. 3 ). These results not only support the view that p41-ARC levels affect FA dimensions and dynamics, but they also suggest that p41-ARC is the variant that is incorporated within the Arp2/3 complex. Taken together these results suggest that vinculin and p41-ARC might alternatively associate with the Arp2/3 core subunits, and, as a consequence, suppression of p41-ARC expression enables vinculin to bind more efficiently to the core components, thus enhancing their recruitment to FAs. To test this possibility, we directly compared Arp2 levels in FAs in p41-ARC knockdown cells with those found in control cells, as shown in Fig. 6a . p41-ARC knockdown indeed induced a major increase in Arp2 levels in FAs as compared with untreated cells, in which the labelling was broadly distributed throughout the lamellipodium, and their association with FAs was typically weak and non-uniform. However, this effect was relatively unpunctuated, likely due to the vast excess (~30-fold) of the classical Arp2/3 pool, relative to the Vin-Arp and Vin-αAct-Arp in HeLa cells ( Fig. 7a,b ). Nevertheless, these observations support the view that, on depletion of p41-ARC, the association of vinculin with the Arp2/3-nucleating core increases, thus promoting recruitment of the complex to FAs. 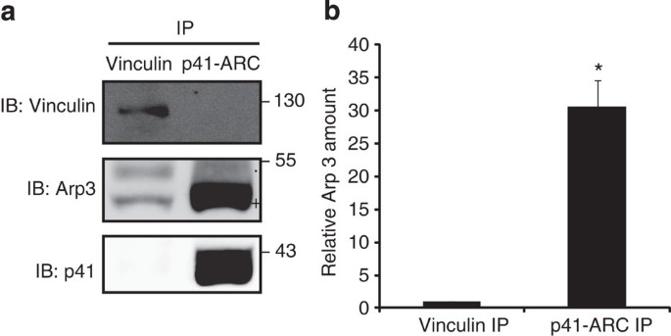Figure 7: The Vin-Arp hybrid complexes have low abundance in comparison with the intact Arp2/3 in HeLa cells. (a) Immunoprecipitation of vinculin and p41-ARC. The plus indicates Arp3 and the dot indicated IgG heavy chain. The original western blot is presented inSupplementary Fig. 5d. (b) Quantification of Arp3 band intensity of CO-IP from two independent experiments. *P<0.05,P-values were calculated by a two-tailed Studentt-test, error bars are ±s.d. Figure 7: The Vin-Arp hybrid complexes have low abundance in comparison with the intact Arp2/3 in HeLa cells. ( a ) Immunoprecipitation of vinculin and p41-ARC. The plus indicates Arp3 and the dot indicated IgG heavy chain. The original western blot is presented in Supplementary Fig. 5d . ( b ) Quantification of Arp3 band intensity of CO-IP from two independent experiments. * P <0.05, P -values were calculated by a two-tailed Student t -test, error bars are ±s.d. Full size image To further assess this hypothesis, biochemically, we compared the relative amounts of Arp2/3 subunits that coimmunoprecipitate with vinculin in p41-ARC knockdown and in control cells. The results of this experiment ( Fig. 6b,c ) indicated that in cells transfected with p41-ARC siRNA, vinculin-bound Arp3 levels are more than twofold higher than those detected in cells transfected with RNA-induced silencing complex-free (RISC) siRNA. In addition, when an antibody directed against p41-ARC was used to probe the vinculin co-IP in both control and p41-ARC knockdown cells, no protein could be detected in either, even though it was clearly detected in the original cell lysate. This finding corroborates our proposal that p41-ARC is absent from the Vin-Arp hybrid complex. Moreover, if indeed p41-ARC controls the alternative targeting of Arp2/3 to either FAs or lamelipodia, knockdown of vinculin should result in stronger association of Arp2/3 with lamellipodia. To examine this idea we utilized H1299 cells, which unlike the relatively immobile HeLa cells are known to be motile, presenting a clearly visible lamellipodium. Indeed, knockdown of p41-ARC induced FA growth and apparent contraction of the cell edge ( Supplementary Fig. 4a ), while knockdown of vinculin resulted in the formation of smaller adhesions, accompanied by intensification of the leading edge ( Supplementary Fig. 4b ). These results are in line with the idea that p41-ARC and vinculin form alternative complexes with the Arp2/3 core components, and that the interaction of these proteins with the core differentially regulates the localization of Arp2/3-dependent actin polymerization. This study reveals a new class of ‘hybrid’ Arp2/3 complexes, containing vinculin, or vinculin plus α-actinin, which are specifically targeted to FAs and play a key role in FA development. Previous studies have shown that actin polymerization takes place in FAs and implicated the two major actin nucleation systems, namely Arp2/3 and formins, in this process [26] , [38] . Arp2/3 components were shown to be associated with integrin adhesions [10] , [18] , [38] ; moreover, it was proposed that the Arp2/3 complex is recruited into FAs by vinculin [38] and/or FAK [39] . Nevertheless, the mechanism whereby the Arp2/3 complex becomes anchored to FA sites is still unknown. The broad assumption is that it is the classical, 7-subunit Arp2/3 that associates with FAs and nucleates actin polymerization in them. The results presented herein provide new and surprising insights into the role of Arp2/3 in FA formation as well as into the mechanisms underlying the subcellular targeting of Arp2/3-driven actin-nucleating activity. We have shown here that vinculin (alone, or together with α-actinin) forms stable complexes with the core subunits of Arp2/3 (Arp2, Arp3 and p34-ARC, with or without p21-ARC, respectively). We assume that one or both of these complexes correspond to the vinculin-Arp2/3 complex described by DeMali et al. [38] Moreover, we demonstrate that knockdown of one of the components of Arp2/3, namely p41-ARC, which is absent from the hybrid complexes, markedly increases the size of FAs and their associated stress fibres ( Fig. 5a,b ), as well as the levels of these complexes in cells ( Fig. 6b,c ) and within FAs ( Fig. 6a ). Furthermore, we show that overexpression of p41-ARC leads to the opposite effect, namely suppression of FA formation ( Fig. 5d,e , and Supplementary Fig. 3 ). These findings support the view that p41-ARC and vinculin replace each other in their binding to the Arp2/3 core components; in the absence of the former, the cellular levels of vinculin-Arp2/3 hybrid complexes, as well as their recruitment to FA sites, increase, enhancing the local nucleation of actin and, consequently, the growth of FAs and the associated stress fibres. This scenario is in line with the study of DeMali et al. [38] , suggesting the involvement of vinculin in recruiting Arp2/3 to FAs. In our MS-based efforts to decompose the intact Arp2/3 and elucidate its structural properties, we used relatively harsh experimental conditions, both in solution (by using denaturing conditions) and in the gas phase (by increasing the accelerating voltage); nevertheless, Arp2/3 proved to be a remarkably stable complex. Only p16-ARC, p21-ARC and p34-ARC were dissociated from the complex during tandem MS, even after prolonged incubation times with 2 M urea or 10 mM imidazole, while Arp2 dissociation was induced only following incubation at high concentrations of potassium iodide ( Supplementary Fig. 1 ). p41-ARC, however, was not expelled from the complex under neither of the experimental conditions. Moreover, it is important to note that we could not produce the Vin-Arp hybrid complex by mixing purified vinculin and Arp2/3. Taking together these observations and knowledge from previous studies, which point to the stability of the Arp2/3 complex [49] , it is tempting to speculate that the formation of the vinculin hybrid complexes occurs at the assembly stage, rather than a result of subunit exchange between vinculin and the classical (seven-subunit) complex. We therefore assume that the biogenesis of the Arp2/3 assemblies occur at the coexpression and coassembly levels. On the basis of the results, presented here, we propose a new model for site-specific actin nucleation by Arp2/3. We suggest that Arp2/3 is composed of two structural and functional modules ( Fig. 8 ). The first, composed of Arp2, Arp3, p34-ARC and possibly p21-ARC, is the nucleation module, responsible for actin polymerization. The second is an ‘anchoring module’, consisting of p16-ARC, p20-ARC and p41-ARC, that localizes the nucleation core on an existing actin filament, thus inducing branching polymerization. We suggest that this anchoring domain can be interchanged with other proteins, such as vinculin, that can direct the actin-nucleating activity to other subcellular sites such as FAs. The mechanism underlying the specification of the localization of the Arp2/3 core remains unclear, although it could involve up-or downregulation of the levels of competing localizing molecules (as demonstrated in this study, when the Arp2/3 core was directed to FAs, following p41-ARC knockdown). 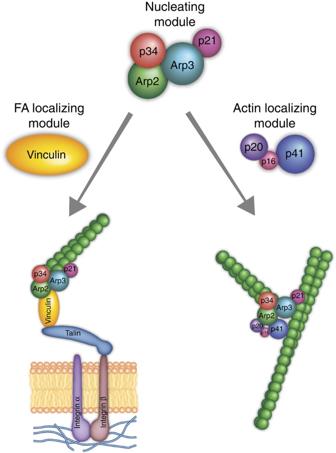Figure 8: The modular structure of the Arp2/3 complex. The functional nucleating module of the complex is composed of Arp2, Arp3 and p34-ARC, with or without p21-ARC. This core unit is then coupled with an anchoring module, either composed of vinculin, which targets the complex to FAs, or p20-ARC, p16-ARC and p41-ARC, which direct the complex to actin-branching sites. Figure 8: The modular structure of the Arp2/3 complex. The functional nucleating module of the complex is composed of Arp2, Arp3 and p34-ARC, with or without p21-ARC. This core unit is then coupled with an anchoring module, either composed of vinculin, which targets the complex to FAs, or p20-ARC, p16-ARC and p41-ARC, which direct the complex to actin-branching sites. Full size image Within that context, it might be interesting to examine whether downregulation of p21-ARC (which is missing from the vinculin-α-actinin-Arp2/3 complex) might enhance the association of α-actinin with the functional core of the Arp2/3 complex. If substantiated as a general mechanism, modulation of the ‘anchorage switching process’ could enable Arp2/3 to selectively activate actin polymerization at different subcellular sites, directed by different anchoring modules. This hypothesis is consistent with previous data regarding the roles of the different Arp2/3 subunits, and the notion in the field that large-scale, multi-subunit structural changes must occur during the activation of the Arp2/3 complex [50] , [51] . p41-ARC itself has multiple functions, associated with different parts of the protein, including prevention of spontaneous nucleation, binding of the WASp VCA domain, propagation of the activation signal to p20-ARC, and binding to actin filaments, all of which suggest that this protein plays an important regulatory role in both the localization and function of the Arp2/3 protein complex [37] , [52] . Moreover, reconstitution experiments have suggested that an Arp2/3 complex lacking p41-ARC and p16-ARC remains active, albeit to a lesser extent [34] . Finally, it is also tempting to speculate about the possible relationships between the adhesion-associated particles described by Patla et al. [16] and the Vin-Arp complexes described herein. The cryo-electron tomography data show the presence of doughnut-shaped particles with a diameter of ~25 nm, located at the interface between the membrane and the short (~50 nm) filaments that associate with the end of a stress fibre [16] . Moreover, immunogold labelling for vinculin of ‘unroofed cells’ indicated that vinculin is either an integral part of the particle or closely associated with it; notably, we commonly observed not one, but two gold particles associated with a single doughnut. Furthermore, the overall dimensions of the Arp2/3 functional complex containing Arp2, Arp3 and p34 are about 10.5 × 10.5 nm 2 , and the dimensions of vinculin are approximately 11.5 × 11.5 nm 2 . Taking these numbers into account, along with the general arc shape of the Arp2/3 complex, it is easy to imagine an adhesion particle made up of two Arp2/3 nucleation cores anchored in place by a pair of vinculin molecules. While these observations provide little direct information on the overall molecular nature of the adhesion-associated particles, they raise the possibility that the Vin-Arp hybrid complexes might be among them. Experiments addressing this possibility are currently in progress. Protein complex isolation and purification Fresh Chicken gizzards (100 g) were homogenized in a 4-l Waring blender with six bursts at maximum speed in 10 volumes of buffer A (20 mM Tris, 40 mM KCl, 40 mM imidazole, 1 mM dithiothreitol (DTT) and 1 mM PMSF, at pH=7.0). The gizzard suspension was then centrifuged in a Sorvall 5c centrifuge, using the SLA3000 rotor for 10 min at 10,000 g , and supernatant was discarded. The pellet was washed again in the same buffer, and supernatant was discarded following centrifugation. To dissociate the remaining actomyosin fibres, the pellet was resuspended in 1 l of buffer A supplemented with 10 mM ATP and centrifuged again at 16,000 g for 10 min. This step was repeated twice. The supernatant was discarded, and the pellet was then resuspended in 1 l of buffer A at pH=9. The resulting suspension was then mixed at 37 °C for 30 min and centrifuged for 10 min at 16,000 g . The pellet was discarded, and the supernatant was subjected to precipitation using 30% ammonium sulphate saturation levels. The mixture was centrifuged at 20,000 g for 30 min, and the supernatant obtained was subjected to precipitation using 50% salt saturation. Following centrifugation at 20,000 g for 30 min, the pellets from each ammonium sulphate step were collected, resuspended in 20 ml of buffer A and combined together. The sample was then loaded onto a 1.8-l kx50 Sepharose 4B gel filtration column (20 mM Tris; pH=7.4), and proteins eluted at 2 ml min −1 were collected in 15 ml fractions. Selected fractions ( Fig. 1b , fractions 10–31) were combined and injected into a 5-ml FastFlow DEAE column at a flow rate of 5 ml min −1 ; proteins were eluted by means of a stepwise gradient into 1.5 ml fractions. Arp2/3 complexes were eluted with 70 mM NaCl. Four fractions of 1.5 ml were pooled together and concentrated to a final concentration of 5 mg ml −1 and an estimated yield of 1 mg total protein. Microscope image acquisition All images were acquired using a Deltavision Elite (Applied Precision, USA) system mounted on an inverted IX71 microscope (Olympus, Japan) connected to a Photometrics CoolSNAP HQ [2] camera (Roper Scientific, USA). The system was running SoftWorX 6.0. Pictures were taken with an × 100 oil ph3 UIS2 UPlanFLN objective with a numerical aperture of 1.3 and an Olympus UIS2 BFP1 × 60 oil PlanApoN objective with a numerical aperture of 1.42 (Olympus, Japan). Cells were imaged in PBS at 37 °C. For actin staining fluorescein isothiocyanate (FITC)- and tetramethylrhodamine (TRITC)-labelled Phalloidin (Sigma) were used. Secondary antibodies (Jackson Immunoresearch) were labelled with Alexa488 and Cy-3 fluorophores. MS analysis Accurate identification of individual protein subunits was carried out either by MS and MS/MS analysis or by the monolithic-liquid chromatography (LC)-MS approach as described [45] . In brief, the individual subunits were separated using a capillary monolithic column (Pepswift, 5 cm × 500 μm, from Dionex, Sunnyville, California). Proteins (5.6 μg) were separated with a linear gradient ranging from 0 to 100% acetonitrile with 0.05% formic acid and 0.035% trifluoroacetic acid, with a flow rate of 15 μl min −1 for 60 min. The flow was then split into two, using the Nanomate robot (Advion, Ithaca, New York). One fraction was sprayed directly into the QSTAR XL mass spectrometer (Applied Biosystems, Foster City, California) for accurate mass determination of the different subunits, whereas the second fraction was collected into a 96-well plate for sequence identity following tryptic digestion, MS analysis and a database search. Proteomic analysis was performed using an UltiMate 3,000 Capillary/Nano LC System and an LTQ-Orbitrap (Thermo Fisher Scientific, Waltham, Massachusetts). Identification of protein by in-gel trypsin digestion was performed as previously described [45] , [53] . In brief, protein samples were reduced with 10 mM DTT for 1 h at 56 °C and then alkylated with 55 mM Iodoacetamide for 30 min at room temperature. This reaction was then quenched with 10 mM DTT. Samples were then digested with trypsin overnight at 37 °C at enzyme to sample ratio of 1:20. This was followed by partial drying of the samples in a SpeedVac. The resulting peptide mixtures were then diluted in 80% formic acid and quickly diluted 1:10 with water. Peptides were then separated by reverse phase LC and analysed by using an LTQ orbitrap XL operating in positive ion mode and equipped with a nano-ESI source. For native MS analysis, 25 μl of the sample was buffer-exchanged into 0.2–1 M ammonium acetate (pH 7.5), using Micro Biospin 6 columns (Bio-Rad, Hercules, California). MS and tandem MS analyses were carried out on a high mass QSTAR instrument [54] . MS parameters were optimized for the transmission of large non-covalent complexes. Typically, aliquots of 2 μl of solution were electrosprayed from gold-coated borosilicate capillaries prepared in-house, as previously described [55] . In brief, borosilicate glass capillaries (1 mm outer diameter × 0.78 mm inner diameter, from Warner instruments, Cat #G100TF- 4) were individually pulled using a needle puller (Model P-97, Sutter instruments) and placed in a 10-cm glass petri dish. Capillaries then underwent through five repeating cycles of gold coating in a sputter coater (model #EMS550, from EMS) using a predefined program (Argon pressure- 4 psi, vacuum pressure set to 5 × 10 −2 mbar, a current of 45 mA). The following experimental parameters were used during the MS experiments: capillary voltage up to 1,250 V; declustering potential up to 180 V; focusing potential up to 250 V; a second declustering potential of 20 V; collision energy of between 20 and 240 V; and an MCP of 2,350 V. Mass spectra were calibrated externally, using a solution of caesium iodide (100 mg ml −1 ). Data were manually analysed using Waters MassLynx software. Compositions of protein complexes and subcomplexes were assigned using an iterative algorithm, SUMMIT, which calculates all possible combinations of subunits that sum to the mass determined experimentally [47] , a 500 Da error limit was used. Spectra are shown with minimal smoothing. MS and MS/MS analysis were performed on three biological replicas. Cell cultures HeLa cells, originally provided from the Cold Spring Harbor Laboratory, were grown in DMEM (Gibco, Grand Island, New York) containing 10% FCS and PenStrep at 37 °C in a 5% CO 2 -humidified atmosphere. H1299 cells, from ATCC, were grown in RPMI 1640 (Gibco) containing 10% FCS and PenStrep. Immunohistochemistry Cells were washed twice with PBS and sequentially fixed in 3% paraformldehyde (PFA) supplemented with 0.5% Triton X-100, followed by 30 min fixation with 3% PFA only. Plates were then incubated for 1 h at room temperature with the primary antibody of choice (mouse anti-vinculin (Cat #V9131, diluted 1:200) from Sigma, mouse anti-Arp2 (Cat #ab49764 diluted 1:200) from Abcam (Cambridge, England) and rabbit anti-zyxin (generated in-house) and washed several times with large volumes of PBS, followed by an additional 1 h incubation with the secondary antibody (Jackson Immunoresearch, West Grove, Pennsylvania) and phalloidin (Sigma. St Louis, Missouri). The fluorescent signal was then visualized, using a DeltaVision microscopy system (Applied Precision, Issaquah, Washington). siRNA screen HeLa cells (about 1,500) were seeded onto fibronectin-covered 96-well plates. Twenty-four hours after replating, cells were transfected with siRNA duplexes (Dharmacon, Lafayette, Colorado) at a final concentration of 50 nM, using the Oligofectamine transfection reagent (Invitrogen, Carlsbad, California), and left to grow for an additional 24 h. Serum was then diluted to a final concentration of 3% to prevent overgrowth of cells. Seventy-two hours post transfection, cells were fixed and stained, as described in the previous section. Dharmacon siGenome smartpools were further validated using individual siRNA sequences. Knockdown of Arp3 was confirmed to be positive with the following target sequences: 5′-GGAAUAUACUGCUGAAAUA-3′, 5′-GACCUAGACUUCUUCAUUG-3′ and 5′-UAAAGGAGCGUAUAGUUA-3′. Knockdown of p41-ARC was confirmed to be positive with the following target sequences- 5′-GAGAAUGACUGGUGGGUUU-3′ and 5′-UAGACUCGCUGCACAAGAA-3′. H1299 cells (~3,000) were transfected with the siRNA duplexes using the DharmaFect 2 (Dharmacon) transfection reagent. 16 h post transfection, the growth media was replaced and cells were left to grow for two more days. Coimmunoprecipitation HeLa cells (~300,000) were seeded onto 10-cm fibronectin-coated plates, and the transfection method described above was rescaled accordingly. Seventy-two hours post transfection, cells were harvested and placed in a buffer containing 20 mM HEPES, 150 mM NaCl, 10% glycerol, 1% Triton X-100 and 1 mM EGTA supplemented with protease inhibitors. The cell lysate was left on ice for 15 min and then centrifuged at 12,000 g for 20 min at 4 °C. The supernatant was removed and placed in a separate tube; 500 μg of each sample was then supplemented with 2 μg of mouse- (Cat #V9264) and rabbit-derived anti-vinculin (Cat #V4139) antibodies (Sigma-Aldrich) or 2 μg of rabbit-derived anti-p41-ARC (Abcam, Cat #ab99314), and left in gentle rotation overnight. Agarose-conjugated protein A/G beads (20 μl) (Santa Cruz, Dallas, Texas) were then added for an additional 1 h, washed several times with the lysis buffer and finally boiled in sample buffer for 5 min. Proteins were separated in a 15% SDS gel, transferred to a nitrocellulose membrane and blotted with antibodies raised against vinculin (from Sigma, Cat #V9264, diluted 1:2,000), p16 (Abcam, Cat #ab51234, diluted 1:1,000) and Arp3 (Abcam, Cat #ab49671, diluted 1:2,000). As non-specific control, we used mouse monoclonal anti-Flag (Sigma #F3165) and mouse anti-Arp3 (Santa Cruz, #sc136279, Abcam,Cat #ab49671). Overexpression of p41-ARC variants A and B HeLa cells (about 5,000) were seeded onto a fibronectin-coated 96-well plate and transfected with 0.25 μg of SOP2HS-pRK5myc (Arpc1a) plasmid or p41-ARC-pRK5myc (Arpc1b), utilizing the JetPEI transfection reagent (Polyplus, New York). Twenty-four hours post transfection, cells were fixed and stained as described. Plasmids were a generous gift from Professor Laura Machesky (University of Glasgow). How to cite this article: Chorev, D. S. et al. Regulation of focal adhesion formation by a vinculin-Arp2/3 hybrid complex. Nat. Commun. 5:3758 doi: 10.1038/ncomms4758 (2014).